The pseudogene TUSC2P promotes TUSC2 function by binding multiple microRNAs Various non-coding regions of the genome, once presumed to be ‘junk’ DNA, have recently been found to be transcriptionally active. In particular, pseudogenes are now known to have important biological roles. Here we report that transcripts of the two tumour suppressor candidate-2 pseudogenes (TUSC2P), found on chromosomes X and Y, are homologous to the 3′-UTR of their corresponding protein coding transcript, TUSC2. TUSC2P and the TUSC2 3′-UTR share many common miRNA-binding sites, including miR-17, miR-93, miR-299-3p, miR-520a, miR-608 and miR-661. We find that ectopic expression of TUSC2P and the TUSC2 3′-UTR inhibits cell proliferation, survival, migration, invasion and colony formation, and increases tumour cell death. By interacting with endogenous miRNAs, TUSC2P and TUSC2 3′-UTR arrest the functions of these miRNAs, resulting in increased translation of TUSC2. The TUSC2P and TUSC2 3′-UTR could thus be used as combinatorial miRNA inhibitors and might have clinical applications. Recently, there has been an increased interest surrounding the functions of non-coding RNA (ncRNA) transcripts. The term ncRNA is given to functional RNA molecules that are not translated to protein. Initially, non-translated regions of the genome were considered ‘junk DNA’ based on the fact that they did not code for proteins and were thus thought to serve no purpose. However, their importance has been revealed in recent years. For example, ncRNAs can regulate microRNA (miRNA) activities. miRNAs are single-stranded RNAs of 18–24 nucleotides in length and are generated from endogenous transcripts [1] , [2] . miRNAs can function as guide molecules in post-transcriptional gene repression through partial binding to the 3′-untranslated region (UTR) [3] . By silencing mRNA targets, miRNAs have been shown to have central roles in physiological and pathological conditions [4] , [5] , [6] . On the other hand, we have previously found that the expression of 3′-UTRs can regulate the function of endogenous miRNAs [7] , [8] , [9] . The 3′-UTR has many functions; it has been known to be involved in messenger RNA (mRNA) nuclear transport, cellular localization, stability and translational efficiency [10] , [11] . These functions are mediated by the presence of several regulatory sequences in the 3′-UTR. These regulatory sequences include the polyadenylation signal, which marks the site of cleavage of the mRNA transcript 30 nt downstream of the signal; binding sites for AU-rich element binding proteins, which can stabilize or destabilize the mRNA depending on the protein; and binding sites for miRNAs [10] , [12] . Interestingly, it has been reported that the 3′-UTRs can be subject to alternative splicing [13] . This finding leads to the idea that splicing occurs in order for the 3′-UTR to escape miRNA regulation under different biological circumstances. However, this idea needs to be further investigated. Our laboratory has been investigating the role and function of the 3′-UTR in relation to miRNAs. It is our hypothesis that overexpression of the 3′-UTR could attract and bind endogenous miRNAs. This would cause the liberation of endogenous 3′-UTRs, whose mRNAs would then be available for translation. Subsequently, there would be an increase in the protein levels of these genes. We initially reported this in Lee et al. [8] , where we found altered cell morphology and increased cell–cell adhesion after the introduction of the exogenous 3′-UTR of versican. This function was due to the ability of the 3′-UTR of versican to antagonize miR-199a-3p functions. One activity of miR-199a-3p was to regulate the expression of two extracellular matrix proteins, versican and fibronectin, which resulted in enhanced cell–cell adhesion and organ adhesion. Furthermore, the versican 3′-UTR overexpression has been found to reduce the steady-state expression of miR-199a-3p [14] . We expanded our research in this field with the investigation of the 3′-UTRs of nephronectin and CD44. We reported that the nephronectin 3′-UTR directed the differentiation rates of MC3T3-E1 cells [15] . Because of binding of endogenous miR-378 and the subsequent increase in GALNT7 expression, the 3′-UTR of nephronectin supported nodule formation and osteoblast differentiation, increasing nephronectin glycosylation and protein secretion. In Jeyapalan et al. [7] , the CD44 3′-UTR was introduced into the MT-1 human breast cancer cell line. It was found that there was a decreased rate of cell proliferation and cell survival, whereas an increased amount of endothelial cell activities and angiogenesis was found. These phenotypic characteristics can be explained owing to the involvement of three miRNAs (miR-216a, miR-330 and miR-608) binding to both the CDC42 and CD44 3′-UTRs. The introduction of the exogenous 3′-UTR of CD44 resulted in the increased protein translation of CDC42 and CD44, both of which are important in cell cycle regulation. We have also reported that the 3′-UTRs of CD44, FN and Col1a1 have multiple miRNAs in common, which increase the metastasis and invasive characteristics of MB231 CD44 3′-UTR-overexpressing cells [16] . Here we continue the investigation of exogenous 3′-UTR overexpression with the TUSC2 3′-UTR. Tumour suppressor candidate-2 ( TUSC2 ), also known as Fus-1 , is a novel tumour suppressor gene that functions as a ‘gatekeeper’ in the molecular pathogenesis of cancer. It was initially identified as part of a study analysing frequent deletions in the short arm of chromosome 3p, which occurs in a wide variety of human cancers, especially of the breast and lung [17] , [18] , [19] . Owing to its recent discovery, very little is known about TUSC2. However, it has been shown to function as a potent proapoptotic factor and has been identified to be involved in the release of cytochrome c from the inner membrane of the mitochondria [20] . Our laboratory previously showed that miR-378 was able to downregulate TUSC2 and Sufu translation. Overexpression of miR-378 resulted in increased cell survival, angiogenesis and tumour growth [4] . While analysing the sequence of the TUSC2 3′-UTR, we identified a sequence with 89% homology to the TUSC2 3′-UTR using the Basic Local Alignment Search Tool as a potential pseudogene of TUSC2 (TUSC2 pseudogene, or TUSC2P). In this study, we exogenously overexpressed TUSC2P and the TUSC2 3′-UTR in breast carcinoma cell lines and found that ectopic expression of TUSC2P and the TUSC2 3′-UTR inhibited cancer cell activities by regulating miRNA functions. Therefore, TUSC2P and the TUSC2 3′-UTR might be used as combinatorial miRNA inhibitors for potential clinical applications. TUSC2P and TUSC2 3′-UTR function as competing endogenous RNAs When analysing the sequence of the TUSC2 3′-UTR, we found that there was one pseudogene of TUSC2, named TUSC2P, expressed by chromosome Y, which shared 99% with a sequence found in chromosome X ( Fig. 1a ). The sequence expressed by the pseudogene TUSC2P from chromosome Y shared 89% homology with the 3′-UTR of TUSC2. Interestingly, many miRNAs were found to have common binding sites for all three sequences, including miR-661, miR-299-3p, miR-93, miR-17, miR-608 and miR-502 ( Fig. 1a ). In particular, the miRNA binding sites were identical to the sequence found in chromosome X and the pseudogene in chromosome Y. Among these miRNAs, some of them displayed more than one potential binding site. Notably, miR-608 displayed four potential binding sites in all three sequences. 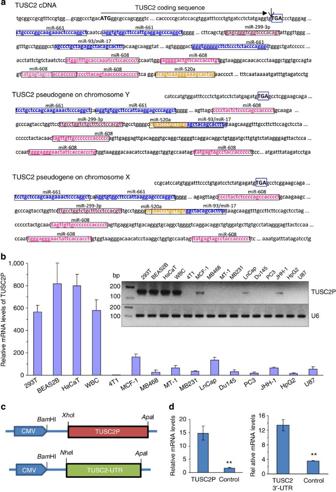Figure 1: Expression of theTUSC2Ppseudogene. (a) Analysis of miRNA targeting the 3′-UTR of TUSC2 and pseudogene TUSC2P on chromosome Y and chromosome X. (b) Expression of TUSC2P was analysed in different cancer and non-cancer cell lines by real-time PCR. The cancer cell lines had a decreased amount of TUSC2P mRNA compared with the non-cancer cell lines. The inset represents bands of reverse transcription–PCR of these cell lines;n=4, error bar, s.d. (c) TUSC2P and TUSC2 3′-UTR were cloned and inserted into pcDNA3.1 plasmid, downstream of the cytomegalovirus promoter, producing the TUSC2P and TUSC2-UTR constructs. (d) Total RNA isolated from 4T1 cells stably transfected with TUSC2P, TUSC2-UTR and control vector were analysed by real-time PCR. The TUSC2P-transfected cells had a fourfold increase compared with the endogenous TUSC2P levels in the cells. The TUSC2-UTR-transfected cells had approximately a threefold increased expression of TUSC2 compared with the control cells;n=3, **P<0.01 analysed byt-test, error bar, s.d. Figure 1: Expression of the TUSC2P pseudogene. ( a ) Analysis of miRNA targeting the 3′-UTR of TUSC2 and pseudogene TUSC2P on chromosome Y and chromosome X. ( b ) Expression of TUSC2P was analysed in different cancer and non-cancer cell lines by real-time PCR. The cancer cell lines had a decreased amount of TUSC2P mRNA compared with the non-cancer cell lines. The inset represents bands of reverse transcription–PCR of these cell lines; n =4, error bar, s.d. ( c ) TUSC2P and TUSC2 3′-UTR were cloned and inserted into pcDNA3.1 plasmid, downstream of the cytomegalovirus promoter, producing the TUSC2P and TUSC2-UTR constructs. ( d ) Total RNA isolated from 4T1 cells stably transfected with TUSC2P, TUSC2-UTR and control vector were analysed by real-time PCR. The TUSC2P-transfected cells had a fourfold increase compared with the endogenous TUSC2P levels in the cells. The TUSC2-UTR-transfected cells had approximately a threefold increased expression of TUSC2 compared with the control cells; n =3, ** P <0.01 analysed by t -test, error bar, s.d. Full size image To examine whether or not the pseudogene was transcribed, we performed reverse transcription–PCR and real-time PCR, confirming that the pseudogene was transcribed into RNA in different cells lines ( Fig. 1b ). Interestingly, results showed high levels of TUSC2P mRNA expression in normal cells, including human white blood cells, human keratinocyte cell line (HaCaT) and human bronchial epithelial cell line (BEAS-2B). Conversely, there was low expression in cancer cells, including human breast cancer cell lines (MDA-MB231, MB468 and MT-1), a human glioblastoma cell line (U87) and a mouse breast cancer cell line (4T1). To study the effects of TUSC2P on regulating miRNA functions, we cloned TUSC2P into the pcDNA3.1 vector ( Fig. 1c ). The mouse and human mammary carcinoma cell lines, 4T1 and MB231, were stably transfected with the TUSC2 3′-UTR and TUSC2P expression constructs. A control cell line was established with the stable transfection of an empty pcDNA3.1 vector. MDA-MB-231 and 4T1 cells were also stably transfected with the coding region of TUSC2 (TUSC2 coding). Expression of TUSC2-UTR or TUSC2P was analysed by real-time PCR. The RNA levels of TUSC2P and TUSC2-UTR in the TUSC2P- and TUSC2-UTR-transfected cells were higher than those of the control and TUSC2 coding, which displayed endogenous levels of TUSC2P and TUSC2-UTR expression ( Fig. 1d and Supplementary Fig. S1a ). This confirmed that the TUSC2P and TUSC2-UTR were being expressed from the TUSC2P and TUSC2-UTR plasmids in our stably transfected cell lines. A series of functional assays were performed in 4T1 cells transfected with TUSC2-UTR, TUSC2P and control cells. Cells transfected with TUSC2-UTR and TUSC2P displayed decreased survival rates ( Fig. 2a ) but increased apoptosis ( Fig. 2b ) compared with the control. In cell migration assay, the TUSC2P- and TUSC2-UTR-transfected cells had reduced rates of migration compared with the control ( Fig. 2c ). When the cells were placed on Matrigel-coated transwell chambers, the control cells invaded through the Matrigel and membrane pores, spreading out on the underside of the membrane significantly more than the TUSC2P and TUSC2-UTR cells ( Fig. 2d ). In addition, MB-231 cells were transfected with TUSC2P, TUSC2-UTR, a construct expressing the TUSC2 coding sequence and a control vector. Expression of these constructs decreased cell proliferation ( Supplementary Fig. S1b ) and survival ( Supplementary Fig. S1c ) compared with the control. Consistent with this was the increased apoptosis when the cells were cultured in serum-free medium ( Supplementary Fig. S1d,e , upper panel) or treated with H 2 O 2 ( Supplementary Fig. S1e , lower panel). 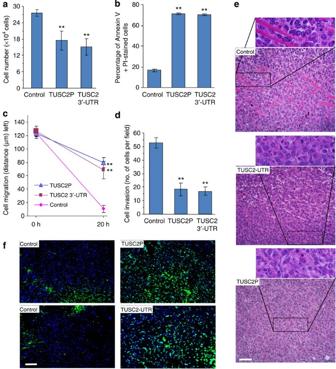Figure 2: TUSC2P and TUSC2 3′-UTR can function as competing endogenous RNAs (ceRNAs). (a) The TUSC2P, TUSC2-UTR and control 4T1 cells were maintained in tissue culture dishes in serum-free conditions. Surviving cells were collected and counted after 8 days. The TUSC2P and TUSC2-UTR cells had a decreased rate of survival;n=3, **P<0.01 analysed byt-test, error bar, s.d. (b) The cells were cultured in serum-free conditions for 5 days, followed by apoptosis analysis. After being stained with Annexin V and PI, the cells were analysed by flow cytometry. The TUSC2P- and TUSC2-UTR-transfected cells had larger populations of apoptotic and necrotic cells (Annexin V positive, PI positive and Annexin V, PI positive) compared with the control cells;n=3, **P<0.01 byt-test, error bar, s.d. (c) Migration rates were monitored using scratch assay. It was found that the TUSC2P- and TUSC2-UTR-transfected 4T1 cells had a slower rate of migration compared with the control cells. **P<0.01 byt-test, error, s.d.,n=10. (d) Cell invasion was examined using Matrigel-coated transwell chambers. When cells were placed in the chambers, the TUSC2P and TUSC2-UTR cells travelled slower through the Matrigel and membrane pores, and spread out on the underside of the membrane significantly less than the control cells;n=5, **P<0.01 byt-test, error bar, s.d. (e) Haematoxylin and eosin staining was performed in tumours formed by injecting TUSC2-UTR, TUSC2P and control 4T1 cells into mice. Evidence of invasive tissues could be seen in the control tumours. However, it was absent in the TUSC2P and TUSC2-UTR tumours. Scale bar, 50 μm. (f) TdT-mediated dUTP nick end labelling staining was performed to observe the apoptotic cells in the tumour sections. Tumours formed by the TUSC2P- and TUSC2-UTR-transfected cells displayed an increased amount of apoptotic cells than the control. Scale bar, 50 μm. Figure 2: TUSC2P and TUSC2 3′-UTR can function as competing endogenous RNAs (ceRNAs). ( a ) The TUSC2P, TUSC2-UTR and control 4T1 cells were maintained in tissue culture dishes in serum-free conditions. Surviving cells were collected and counted after 8 days. The TUSC2P and TUSC2-UTR cells had a decreased rate of survival; n =3, ** P <0.01 analysed by t -test, error bar, s.d. ( b ) The cells were cultured in serum-free conditions for 5 days, followed by apoptosis analysis. After being stained with Annexin V and PI, the cells were analysed by flow cytometry. The TUSC2P- and TUSC2-UTR-transfected cells had larger populations of apoptotic and necrotic cells (Annexin V positive, PI positive and Annexin V, PI positive) compared with the control cells; n =3, ** P <0.01 by t -test, error bar, s.d. ( c ) Migration rates were monitored using scratch assay. It was found that the TUSC2P- and TUSC2-UTR-transfected 4T1 cells had a slower rate of migration compared with the control cells. ** P <0.01 by t -test, error, s.d., n =10. ( d ) Cell invasion was examined using Matrigel-coated transwell chambers. When cells were placed in the chambers, the TUSC2P and TUSC2-UTR cells travelled slower through the Matrigel and membrane pores, and spread out on the underside of the membrane significantly less than the control cells; n =5, ** P <0.01 by t -test, error bar, s.d. ( e ) Haematoxylin and eosin staining was performed in tumours formed by injecting TUSC2-UTR, TUSC2P and control 4T1 cells into mice. Evidence of invasive tissues could be seen in the control tumours. However, it was absent in the TUSC2P and TUSC2-UTR tumours. Scale bar, 50 μm. ( f ) TdT-mediated dUTP nick end labelling staining was performed to observe the apoptotic cells in the tumour sections. Tumours formed by the TUSC2P- and TUSC2-UTR-transfected cells displayed an increased amount of apoptotic cells than the control. Scale bar, 50 μm. Full size image The tumorigenic potential of TUSC2P and TUSC2-UTR-transfected 4T1 cells was tested in BALB/c mice. Although there was no significant difference in tumour size when tumours were excised from the mice and subjected to haematoxylin and eosin staining, the control tumours showed histological evidence of increased invasiveness. Mouse muscle tissue was surrounded by tumour tissue, which was not present in the TUSC2-UTR and TUSC2P tumours ( Fig. 2e ). Furthermore, the TUSC2-UTR and TUSC2P tumour sections exhibited more apoptotic cells than the control tumour sections when subject to TdT-mediated dUTP nick end labelling staining ( Fig. 2f ). Targets of miRNAs interacting with TUSC2 and TUSC2P To examine whether TUSC2P and TUSC2-UTR exerted their biological functions by modulating miRNAs that interacted with these two sequences, we analysed the potential targets of these miRNAs. By in silico analysis, we found that the 3′-UTRs of tissue inhibitor of metalloproteinases-2 (TIMP2) and TIMP3 could also bind many of these miRNAs ( Fig. 3a ). It is known that both TIMP2 and TIMP3 are involved in cell migration, adhesion and metastasis [21] , [22] , [23] . We hypothesized that overexpression of the non-coding transcripts, TUSC2P or TUSC2 3′-UTR, was able to antagonize multiple miRNAs, thus relieving translational inhibition of the mRNAs of TUSC2, TIMP2 and TIMP3 ( Fig. 3a ). Comparing the sequences of these miRNAs with TUSC2-UTR ( Fig. 3b ), TUSC2P ( Fig. 3c ), TIMP2 and TIMP3 ( Fig. 3d ) showed that these four mRNAs were highly homologous in miRNA binding sites. 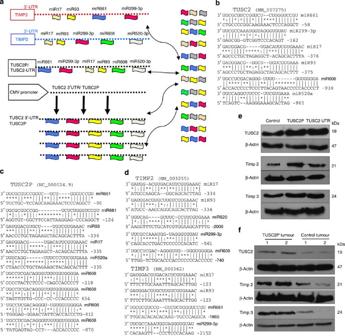Figure 3: Targeting of TUSC2 and TIMP2/3 by miRNAs. (a) We hypothesized that the TUSC2P/TUSC2-UTR would attract endogenous miR-17, miR-93, miR-299-3p, miR-520a, miR-608 and miR-661, thus freeing TUSC2, TIMP2 and TIMP3 mRNAs to be available for translation. (b) Computation analysis of the TUSC2 showed potential binding sites for miR-93, miR-299-3p, miR-520a, miR-17, miR-608 and miR-661. (c) Computation analysis of the TUSC2P showed potential binding sites for miR-93, miR-17, miR-520a, miR-608 and miR-661. (d) Computation analysis of TIMP2 3′-UTR (upper) and TIMP3 (lower) 3′-UTRs revealed binding sites for miR-17, miR-93, miR-299-3p, miR-608 and miR-661. (e) Protein lysates were prepared from TUSC2P-, TUSC2-UTR- and vector-transfected cells and subjected to western blot analysis probed with anti-TUSC2, anti-TIMP2 and anti-TIMP3 antibodies. There was elevated expression of TUSC2, TIMP2 and TIMP3 in the TUSC2P and TUSC2-UTR cells compared with the control cells. Detection of β-actin on the same membranes served as a loading control. (f) Protein lysates were prepared from TUSC2P and control tumours, and subject to western blot analysis and probed with anti-TUSC2, anti-TIMP2 and anti-TIMP3 antibodies. TUSC2, TIMP2 and TIMP3 were upregulated in the TUSC2P tumours. Figure 3: Targeting of TUSC2 and TIMP2/3 by miRNAs. ( a ) We hypothesized that the TUSC2P/TUSC2-UTR would attract endogenous miR-17, miR-93, miR-299-3p, miR-520a, miR-608 and miR-661, thus freeing TUSC2, TIMP2 and TIMP3 mRNAs to be available for translation. ( b ) Computation analysis of the TUSC2 showed potential binding sites for miR-93, miR-299-3p, miR-520a, miR-17, miR-608 and miR-661. ( c ) Computation analysis of the TUSC2P showed potential binding sites for miR-93, miR-17, miR-520a, miR-608 and miR-661. ( d ) Computation analysis of TIMP2 3′-UTR (upper) and TIMP3 (lower) 3′-UTRs revealed binding sites for miR-17, miR-93, miR-299-3p, miR-608 and miR-661. ( e ) Protein lysates were prepared from TUSC2P-, TUSC2-UTR- and vector-transfected cells and subjected to western blot analysis probed with anti-TUSC2, anti-TIMP2 and anti-TIMP3 antibodies. There was elevated expression of TUSC2, TIMP2 and TIMP3 in the TUSC2P and TUSC2-UTR cells compared with the control cells. Detection of β-actin on the same membranes served as a loading control. ( f ) Protein lysates were prepared from TUSC2P and control tumours, and subject to western blot analysis and probed with anti-TUSC2, anti-TIMP2 and anti-TIMP3 antibodies. TUSC2, TIMP2 and TIMP3 were upregulated in the TUSC2P tumours. Full size image TIMP2 and TIMP3 are proteins that are critical for the inhibition of matrix metalloproteinases, a group of proteases involved in the extracellular matrix remodelling of tissues [24] , [25] , [26] . We hypothesized that an increase in TUSC2P and TUSC 3′-UTR levels should be followed by an increase in TUSC2, TIMP2 and TIMP3 protein levels, as miRNAs would bind to the overexpressed TUSC2P and TUSC 3′-UTR, freeing the endogenous mRNAs of TUSC2, TIMP2 and TIMP3. This was confirmed by western blotting using cell lysates from TUSC2P, TUSC2-UTR and control cells. Indeed, we detected elevated expression of TUSC2, TIMP2 and TIMP3 in the TUSC2P and TUSC2-UTR cells but not in the control cells ( Fig. 3e ). Tumours created from mice injected with the TUSC2P-transfected 4T1 cells were analysed by western blotting. It was found that the TUSC2P tumours had higher TUSC2, TIMP2 and TIMP3 protein expression levels, as compared with the control tumours ( Fig. 3f ). This increase was also seen by immunostaining of TUSC2P, TUSC2-UTR and control tumours: both TUSC2-UTR and TUSC2P tumours had a higher amount of TUSC2, TIMP2 and TIMP3 expression than the control tumours ( Supplementary Fig. S2a ). We also performed these experiments in MDA-MB-231 cells stably transfected with TUSC2P, TUSC2-UTR and a control vector. Cells transfected with TUSC2P expressed higher levels of TUSC2, TIMP2 and TIMP3 than the control cells ( Supplementary Fig. S2b ). As expected, although transfection with the TUSC2-coding region increased TUSC2 expression, it did not increase TIMP2 and TIMP3 protein levels ( Supplementary Fig. S2c ). Endogenous expression of TUSC2, TIMP2 and TIMP3 was analysed in a number of cancer and non-cancer cell lines. In general, although we did not detect higher mRNA levels of TUSC2 ( Fig. 4a ), TIMP2 ( Fig. 4b ) and TIMP3 ( Fig. 4c ) in cancerous cells, we detected lower levels of these proteins in the cancer cells than in the non-cancerous cell lines, Hek-293T, BEAS2B and HaCaT. We also examined the expression of TUSC2, TIMP2 and TIMP3 in human breast cancer specimens. Although these proteins could be clearly detected in the ductal structures of breast tissues, they were almost undetectable in tumour tissues ( Fig. 4d ). 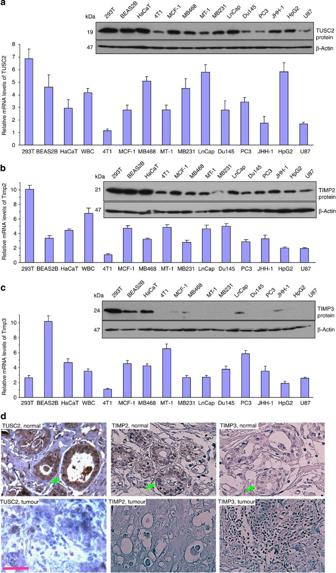Figure 4: Expression of TUSC2 and TIMP2/3 in different cell lines and patient specimens. (a–c) Expression of TUSC2 (a), TIMP2 (b) and TIMP3 (c) were analysed by real-time PCR for mRNA levels and western blotting for protein levels (insets) in different cell lines as indicated;n=4, error bar, s.d. (d) Human breast cancer specimens were probed for expression of TUSC2, TIMP2 and TIMP3. Expression of these molecules was detected in the ductal structures (arrows), but not in the tumour tissues. Scale bar, 50 μm. Figure 4: Expression of TUSC2 and TIMP2/3 in different cell lines and patient specimens. ( a – c ) Expression of TUSC2 ( a ), TIMP2 ( b ) and TIMP3 ( c ) were analysed by real-time PCR for mRNA levels and western blotting for protein levels (insets) in different cell lines as indicated; n =4, error bar, s.d. ( d ) Human breast cancer specimens were probed for expression of TUSC2, TIMP2 and TIMP3. Expression of these molecules was detected in the ductal structures (arrows), but not in the tumour tissues. Scale bar, 50 μm. Full size image Validation of miRNA function The binding of miRNAs to TUSC2P, the 3′-UTRs of TUSC2, TIMP2 and TIMP3 was confirmed by luciferase assay. As indicated in the Supplementary Fig. S3 , we generated five luciferase constructs containing fragments of TIMP2 3′-UTR harbouring binding sites for miR-17, miR-93, miR-299-3p, miR-520-3p and miR-608. Each construct was subject to site-directed mutagenesis, abolishing the miRNA binding activity. We also generated four luciferase constructs containing fragments of TIMP3 3′-UTR harbouring binding sites for miR-17, miR-93, miR-299-3p and miR-661. The binding sites were mutated, resulting in four mutant constructs ( Supplementary Fig. S4 ). As there were many potential miRNA binding sites common in the 3′-UTR of TUSC2 and the pseudogene TUSC2P, we used TUSC2P to validate the effect of each miRNA on binding to TUSC2P. Six miRNAs were tested by generating luciferase constructs and mutant constructs as shown ( Supplementary Fig. S5 ). Each luciferase construct was paired with the corresponding mutant and a construct inserted with a non-related sequence (Luc-G3R) serving as a control. Cells were co-transfected with the corresponding miRNA mimics and one of these constructs, followed by luciferase activity analysis. We found that luciferase activity was significantly repressed in the TUSC2P luciferase constructs when co-transfected with miR-299-3p ( Fig. 5a ), miR-661 ( Fig. 5b ), miR-17 ( Fig. 5c ), miR-93 ( Fig. 5d ), miR-520a ( Fig. 5e ) and miR-608 ( Fig. 5f ). Mutation of the binding site reversed the repression significantly. We also found that luciferase activity was significantly repressed in the TIMP2 constructs when co-transfected with miR-93 ( Fig. 5g ), miR-299-3p ( Fig. 5h ), miR-17 ( Fig. 5i ), miR-608 ( Fig. 5j ) and miR-520a ( Fig. 5k ). Mutation of the binding sites reversed the repressive effect. Similarly, luciferase activity was repressed in TIMP3 constructs when the cells were co-transfected with miR-93 ( Fig. 5l ), miR-299-3p ( Fig. 5m ), miR-17 ( Fig. 5n ) and miR-661 ( Fig. 5o ), and the inhibition was reversed when the binding sites were mutated. 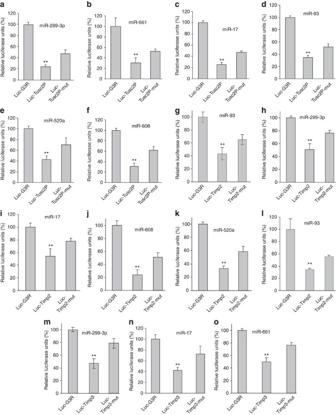Figure 5: Confirmation of TIMP2 and TIMP3 targeting. (a–f) Fragments of TUSC2P harbouring different target sites of miR-299-3p (a), miR-661 (b), miR-17 (c), miR-93 (d), miR-520a (e) and miR-608 (f) were cloned into the luciferase reporter vector pMir-Report. 4T1 cells were co-transfected with one of these miRNAs and the luciferase constructs or a mutant constructs, in which the miRNA target sites were mutated. A non-related fragment of complementary DNA was used as a positive control. Luciferase activity assays indicated that all six miRNAs repressed luciferase activities when it harboured the corresponding TUSC2P fragment, which was reversed when the potential miRNA target site was mutated;n=3, **P<0.01 (between wild type and mutants) byt-test, error bar, s.d. (g–k) The cells were co-transfected with luciferase reporter plasmids for TIMP2 with corresponding miRNAs or a control oligo. In the presence of the targeting UTR, luciferase activities were inhibited, which were significantly elevated when the target sites were mutated;n=3, **P<0.01 (between wild type and mutants) byt-test, error bar, s.d. (l–o) The TIMP3 3′-UTR fragments containing the binding sites for miR-17, miR-93, miR-299-3p and miR-661 were cloned into pMir-Report. Luciferase activity assays indicated that all four miRNAs repressed luciferase activities, which was reversed when the miRNA binding site was mutated;n=3, **P<0.01 (between wild type and mutants) byt-test, error bar, s.d. Figure 5: Confirmation of TIMP2 and TIMP3 targeting. ( a – f ) Fragments of TUSC2P harbouring different target sites of miR-299-3p ( a ), miR-661 ( b ), miR-17 ( c ), miR-93 ( d ), miR-520a ( e ) and miR-608 ( f ) were cloned into the luciferase reporter vector pMir-Report. 4T1 cells were co-transfected with one of these miRNAs and the luciferase constructs or a mutant constructs, in which the miRNA target sites were mutated. A non-related fragment of complementary DNA was used as a positive control. Luciferase activity assays indicated that all six miRNAs repressed luciferase activities when it harboured the corresponding TUSC2P fragment, which was reversed when the potential miRNA target site was mutated; n =3, ** P <0.01 (between wild type and mutants) by t -test, error bar, s.d. ( g – k ) The cells were co-transfected with luciferase reporter plasmids for TIMP2 with corresponding miRNAs or a control oligo. In the presence of the targeting UTR, luciferase activities were inhibited, which were significantly elevated when the target sites were mutated; n =3, ** P <0.01 (between wild type and mutants) by t -test, error bar, s.d. ( l – o ) The TIMP3 3′-UTR fragments containing the binding sites for miR-17, miR-93, miR-299-3p and miR-661 were cloned into pMir-Report. Luciferase activity assays indicated that all four miRNAs repressed luciferase activities, which was reversed when the miRNA binding site was mutated; n =3, ** P <0.01 (between wild type and mutants) by t -test, error bar, s.d. Full size image The miRNAs used in this study were overexpressed in the TUSC2 3′-UTR 4T1 cells to observe the functions of these individual miRNAs. This was also done to confirm the function of these miRNAs in relation to the TUSC2 3′-UTR. TUSC2 3′-UTR 4T1 cells transfected with miR-17, miR-93, miR-299-3p, miR-520-3p, miR-608, miR-661 or a negative control oligo were subject to western blot analysis. There was a repression of TUSC2 levels by the overexpression of these miRNAs as compared with the control ( Fig. 6a ). This confirmed that the TUSC2 3′-UTR was a direct target of these six miRNAs. Furthermore, when the TUSC2P 4T1 cells were transfected with these miRNAs, there was a decrease in the levels of both TIMP2, targeted by miR-17, miR-93, miR-299-3p, miR-520-3p and miR-608, and TIMP3, targeted by miR-17, miR-93, miR-299-3p and miR-661 ( Fig. 6b ). 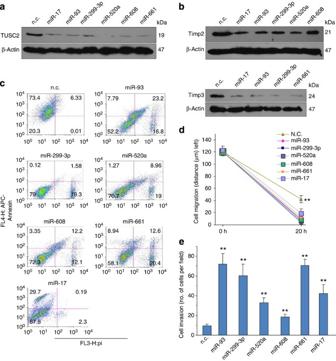Figure 6: Functional analysis of miRNAs targeting TUSC2. (a) Lysates of 4T1 cells transfected with miRNAs were analysed by western blotting. Expression of miR-17, miR-93, miR-299-3p, miR-520a, miR-608 and miR-661 decreased TUSC2 protein levels. β-Actin on the same membranes served as a loading control. (b) The cells transfected with different miRNAs were subject to western blot analysis for expression of TIMP2 and TIMP3. Both TIMP2 and TIMP3 levels decreased in cells transfected with miRNAs as compared with the control oligo. (c) Apoptosis was analysed in cells transfected with different miRNAs. Transfection with the miRNAs decreased apoptosis;n=3, **P<0.01. (d) The migration rate was measured for the miRNA-transfected 4T1 cells. There was an increased amount of cell migration in miRNA-transfected cells compared with control cells;n=10, **P<0.01 byt-test, error bar, s.d. (e) In cell invasion assays, the cells transfected with miR-17, miR-93, miR-299-3p, miR-520a, miR-608 and miR-661 showed drastically increased in the capacity of invasion through the membrane pores compared with the control cells;n=5, **P<0.01 byt-test. Figure 6: Functional analysis of miRNAs targeting TUSC2. ( a ) Lysates of 4T1 cells transfected with miRNAs were analysed by western blotting. Expression of miR-17, miR-93, miR-299-3p, miR-520a, miR-608 and miR-661 decreased TUSC2 protein levels. β-Actin on the same membranes served as a loading control. ( b ) The cells transfected with different miRNAs were subject to western blot analysis for expression of TIMP2 and TIMP3. Both TIMP2 and TIMP3 levels decreased in cells transfected with miRNAs as compared with the control oligo. ( c ) Apoptosis was analysed in cells transfected with different miRNAs. Transfection with the miRNAs decreased apoptosis; n =3, ** P <0.01. ( d ) The migration rate was measured for the miRNA-transfected 4T1 cells. There was an increased amount of cell migration in miRNA-transfected cells compared with control cells; n =10, ** P <0.01 by t -test, error bar, s.d. ( e ) In cell invasion assays, the cells transfected with miR-17, miR-93, miR-299-3p, miR-520a, miR-608 and miR-661 showed drastically increased in the capacity of invasion through the membrane pores compared with the control cells; n =5, ** P <0.01 by t -test. Full size image We examined phenotypic changes of the 4T1 cells transfected with these miRNAs. TUSC2P cells were transfected with the miRNAs or a negative control oligo, followed by Annexin V apoptosis assay. It was found that the miRNA-transfected cells had a decreased amount of cell apoptosis than the control cells ( Fig. 6c ). Migration assays showed that there was an increased rate of cell migration in the miRNA-transfected TUSC2P cells compared with the control TUSC2P cells ( Fig. 6d ). The functions of these miRNAs were further tested by transwell Matrigel invasion assay. Relative to control cells, an increased migratory capacity was observed in cells that were transfected with miR-93, miR-17, miR-299-3p and miR-661 ( Fig. 6e ). In addition, miR-520-3p and miR-608 transfection also resulted in increased invasive capacity; however, the results were not as drastic as in miR-17-, miR-93-, miR-299-3p- and miR-661-transfected cells. Collectively, these results demonstrated that all of miR-17, miR-93, miR-299-3p, miR-520-3p, miR-608 and miR-661 were involved in migration and invasion. Notably, some miRNAs elicited a stronger phenotypic change than others. For example, miR-93 had a stronger effect on cell migration and invasion than the other miRNAs. Our experiments directly confirmed the functions of TUSC2P and TUSC2 3′-UTR in 4T1 cells. Validation of TUSC2P effects As 4T1 cells expressed undetectable levels of TUSC2P and HaCaT cells expressed very high levels of TUSC2P, we analysed the copy number of both TUSC2P and TUSC2 using the method described [27] . In the vector-transfected cells, both 4T1 and HaCaT cells expressed TUSC2, but TUSC2P was expressed only in HaCaT cells ( Fig. 7a ). In both 4T1 and HaCaT, TUSC2P transfection only somewhat upregulated the expression levels of TUSC2P ( Fig. 7b ). The upregulation of TUSC2P was significant in 4T1 cells but not in HaCaT cells, perhaps due to the high background levels of TUSC2P ( Fig. 7c ). 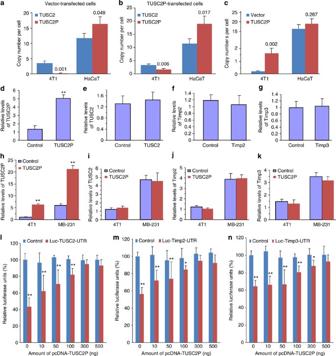Figure 7: Expression of TUSC2P affects activities of TUSC2 and TIMP3. (a,b) Copy number of TUSC2 and TUSC2P was determined in vector- and TUSC2P-transfected cells.P-values are obtained byt-test and shown in the figure;n=3, error bar, s.d. (c) Copy number of TUSC2P was determined in vector- and TUSC2P-transfected cells. Expression of TUSC2P (d), TUSC2 (e), TIMP2 (f) and TIMP3 (g) was analysed in tumours formed by cells transfected with the control vector or TUSC2P. Although TUSC2P levels were promoted in the TUSC2P tumour, there was little difference in the expression of the others;n=3, **P<0.01 byt-test, error bar, s.d. Expression of TUSC2P (h), TUSC2 (i), TIMP2 (j) and TIMP3 (k) was analysed in 4T1 and MDA-MB-231 cells transfected with the control vector or TUSC2P. TUSC2P transfection did not affect expression of TUSC2, TIMP2 and TIMP3;n=3, **P<0.01 byt-test, error bar, s.d. Luciferase constructs for the 3′-UTRs of TUSC2 (l), TIMP2 (m) and TIMP3 (n) were co-transfected with TUSC2P in 4T1 cells. Increased amounts of TUSC2P promoted the activities of the luciferase constructs;n=3, *P<0.05, **P<0.01 byt-test, error bar, s.d. Figure 7: Expression of TUSC2P affects activities of TUSC2 and TIMP3. ( a , b ) Copy number of TUSC2 and TUSC2P was determined in vector- and TUSC2P-transfected cells. P -values are obtained by t -test and shown in the figure; n =3, error bar, s.d. ( c ) Copy number of TUSC2P was determined in vector- and TUSC2P-transfected cells. Expression of TUSC2P ( d ), TUSC2 ( e ), TIMP2 ( f ) and TIMP3 ( g ) was analysed in tumours formed by cells transfected with the control vector or TUSC2P. Although TUSC2P levels were promoted in the TUSC2P tumour, there was little difference in the expression of the others; n =3, ** P <0.01 by t -test, error bar, s.d. Expression of TUSC2P ( h ), TUSC2 ( i ), TIMP2 ( j ) and TIMP3 ( k ) was analysed in 4T1 and MDA-MB-231 cells transfected with the control vector or TUSC2P. TUSC2P transfection did not affect expression of TUSC2, TIMP2 and TIMP3; n =3, ** P <0.01 by t -test, error bar, s.d. Luciferase constructs for the 3′-UTRs of TUSC2 ( l ), TIMP2 ( m ) and TIMP3 ( n ) were co-transfected with TUSC2P in 4T1 cells. Increased amounts of TUSC2P promoted the activities of the luciferase constructs; n =3, * P <0.05, ** P <0.01 by t -test, error bar, s.d. Full size image To examine the effects of TUSC2P, we tested whether the expression of TUSC2P affected levels of other mRNAs in tumours formed by TUSC2P- or vector-transfected cells. Although TUSC2P levels were increased in the TUSC2P tumours ( Fig. 7d ), there was little difference in levels of TUSC2 ( Fig. 7e ), TIMP2 ( Fig. 7f ) or TIMP3 ( Fig. 7g ). To corroborate these results, 4T1 and MB231 cells were transfected with TUSC2P or a control vector. It was found that cells transfected with TUSC2P expressed higher levels of TUSC2P than the control groups ( Fig. 7h ), but there was little difference in the expression of TUSC2 ( Fig. 7i ), TIMP2 ( Fig. 7j ) and TIMP3 ( Fig. 7k ). We then tested the effects of TUSC2P on luciferase constructs harbouring the 3′-UTRs of TUSC2, TIMP2 and TIMP3 in competition assays. It was found that luciferase activity was increased in a dose-dependent manner when the constructs contained the TUSC2-UTR ( Fig. 7l ), TIMP2-UTR ( Fig. 7m ) and TIMP3-UTR ( Fig. 7n ) sequences. To confirm that the phenotypic changes were due to TUSC2P, siRNA sequences were designed to target TUSC2P and to suppress its function. HaCaT and MB231 cells were transfected with these siRNAs, using an unrelated sequence as a control. Western blot analysis was performed and the siRNA-treated HaCaT were found to have decreased TUSC2, TIMP2 and TIMP3 protein levels ( Fig. 8a ). 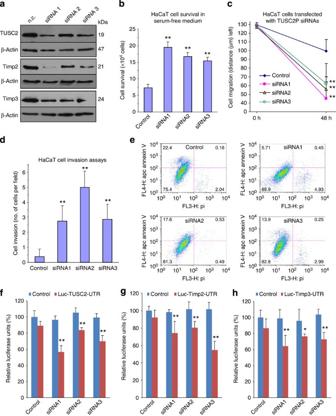Figure 8: Confirmation of TUSC2P effects by siRNA approach. (a) Lysates prepared from the siRNA-treated HaCaT cells were subject to western blot analysis. Levels of TUSC2, TIMP2 and TIMP3 decreased as a result of siRNA targeting TUSC2P. (b) Cell survival was analysed in cells transfected with siRNAs targeting TUSC2P or a control oligo. The TUSC2P siRNA-treated cells survived longer in serum-free medium than the control cells;n=5,P<0.01 byt-test, error bar, s.d. (c) In migration assay, the siRNA-treated cells migrated faster than the cells transfected with a control oligo;n=5, **P<0.01 byt-test, error bar, s.d. (d) In invasion assay, there was an increased amount of the siRNA-treated cells that invaded through the Matrigel compared with the control;n=5, **P<0.01 byt-test, error bar, s.d. (e) Determination of cell apoptosis indicated that less siRNA-treated cells underwent apoptosis than the control cells;n=10. The luciferase constructs of TUSC2 (f), TIMP2 (g) and TIMP3 (h) were co-transfected with siRNA targeting endogenous TUSC2P in HaCaT cells. Silencing TUSC2P decreased luciferase activities;n=5, *P<0.05, **P<0.01 byt-test, error bar, s.d. Figure 8: Confirmation of TUSC2P effects by siRNA approach. ( a ) Lysates prepared from the siRNA-treated HaCaT cells were subject to western blot analysis. Levels of TUSC2, TIMP2 and TIMP3 decreased as a result of siRNA targeting TUSC2P. ( b ) Cell survival was analysed in cells transfected with siRNAs targeting TUSC2P or a control oligo. The TUSC2P siRNA-treated cells survived longer in serum-free medium than the control cells; n =5, P <0.01 by t -test, error bar, s.d. ( c ) In migration assay, the siRNA-treated cells migrated faster than the cells transfected with a control oligo; n =5, ** P <0.01 by t -test, error bar, s.d. ( d ) In invasion assay, there was an increased amount of the siRNA-treated cells that invaded through the Matrigel compared with the control; n =5, ** P <0.01 by t -test, error bar, s.d. ( e ) Determination of cell apoptosis indicated that less siRNA-treated cells underwent apoptosis than the control cells; n =10. The luciferase constructs of TUSC2 ( f ), TIMP2 ( g ) and TIMP3 ( h ) were co-transfected with siRNA targeting endogenous TUSC2P in HaCaT cells. Silencing TUSC2P decreased luciferase activities; n =5, * P <0.05, ** P <0.01 by t -test, error bar, s.d. Full size image The effects of siRNAs on cell phenotypes were then tested. siRNA treatment on TUSC2P cells increased survival compared with the control ( Fig. 8b ). The siRNAs also enhanced migratory ( Fig. 8c ) and invasive capacity ( Fig. 8d ), while reducing cell apoptosis ( Fig. 8e ), compared with the control. To corroborate these results, we treated HaCaT cells with siRNAs targeting endogenous TUSC2P and found that silencing endogenous TUSC2P repressed luciferase activity when the constructs contained either TUSC2-UTR ( Fig. 8f ), TIMP2-UTR ( Fig. 8g ) or TIMP3-UTR ( Fig. 8h ). In MB231 cells, siRNA-1 and siRNA-2 had strong interfering effects, whereas siRNA-3 only weakly decreased the expression of TUSC2, TIMP2 and TIMP3 ( Supplementary Fig. S6a ). We also detected decreased cell apoptosis ( Supplementary Fig. S6b ), but enhanced cell migration ( Supplementary Fig. S6c ) and invasion ( Supplementary Fig. S6d ) in the cells transfected with siRNAs. Thus, the siRNAs that targeted TUSC2P were able to downregulate TUSC2P functions, reversing the observed phenotype. These siRNAs were found to decrease levels of TUSC2P ( Supplementary Fig. S6e ), but had little effect on the expression of TUSC2 ( Supplementary Fig. S6f ), TIMP2 ( Supplementary Fig. S6g ) and TIMP3 ( Supplementary Fig. S6h ). To confirm that the observed transcriptional effects and phenotype of TUSC2P cells were mediated through miRNAs, we treated HaCaT cells with an siRNA targeting Dicer1 to block the miRNA biogenesis pathway. As expected, silencing Dicer1 decreased levels of the miRNAs tested ( Fig. 9a ). As a consequence, silencing Dicer1 increased the expression of TUSC2, TIMP2 and TIMP3 ( Fig. 9b ). Luciferase assays showed that silencing TUSC2P decreased the effects of TUSC2P on promoting luciferase activity, when the construct contained the 3′-UTRs of TUSC2 ( Fig. 9c ), TIMP2 ( Fig. 9d ) and TIMP3 ( Fig. 9e ). However, in the presence of Dicer1 siRNA, the effects of TUSC2P transfection were abolished and we confirmed silencing of TUSC2P even in the presence of Dicer1 siRNA ( Fig. 9f ). 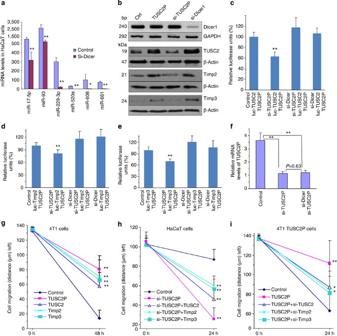Figure 9: Confirmation of TUSC2P functions. (a) HaCaT cells were transfected with an siRNA targeting Dicer1 to block the miRNA biogenesis pathway. Silencing Dicer1 decreased levels of the miRNAs tested;n=4, *P<0.05, **P<0.01 byt-test, error bar, s.d. (b) HaCaT cells were treated with siRNA targeting Dicer1 or TUSC2P followed by reverse transcription–PCR for confirmation of Dicer knockdown and western blot analysis to analyse levels of TUSC2, TIMP2 and TIMP3. Silencing Dicer increased expression of TUSC2, TIMP2 and TIMP3. HaCaT cells were transfected with luciferase constructs of TUSC2 (c), TIMP2 (d) and TIMP3 (e) combined with TUSC2P, siRNA targeting TUSC2P, and/or siRNA targeting Dicer1 followed by luciferase assays. Although silencing TUSC2P decreased luciferase activities, silencing Dicer reversed the effects;n=4, **P<0.01 analysed byt-test, error bar, s.d. (f) HaCaT cells were transfected with TUSC2P siRNA combined with or without Dicer1 siRNA. TUSC2P was silenced even in the presence of Dicer1 siRNA;n=4, **P<0.01 analysed byt-test, error bar, s.d. (g) Transfection of 4T1 cells with TUSC2P, TUSC2, TIMP2 and TIMP3 decreased cell migration;n=4, **P<0.01 analysed byt-test, error bar, s.d. (h) Transfection of HaCaT cells with siRNA targeting endogenous TUSC2P increased cell migration. Combined transfection with TUSC2, TIMP2 or TIMP3 partially, but significantly, reversed the effect of TUSC2P on cell migration;n=4, **P<0.01 analysed byt-test, error bar, s.d. (i) Transfection of 4T1 cells with TUSC2P decreased cell migration, which could be partially, but significantly, reversed by transfection with siRNAs targeting TUSC2, TIMP2 or TIMP3;n=4, *P<0.05, **P<0.01 byt-test, error bar, s.d. Figure 9: Confirmation of TUSC2P functions. ( a ) HaCaT cells were transfected with an siRNA targeting Dicer1 to block the miRNA biogenesis pathway. Silencing Dicer1 decreased levels of the miRNAs tested; n =4, * P <0.05, ** P <0.01 by t -test, error bar, s.d. ( b ) HaCaT cells were treated with siRNA targeting Dicer1 or TUSC2P followed by reverse transcription–PCR for confirmation of Dicer knockdown and western blot analysis to analyse levels of TUSC2, TIMP2 and TIMP3. Silencing Dicer increased expression of TUSC2, TIMP2 and TIMP3. HaCaT cells were transfected with luciferase constructs of TUSC2 ( c ), TIMP2 ( d ) and TIMP3 ( e ) combined with TUSC2P, siRNA targeting TUSC2P, and/or siRNA targeting Dicer1 followed by luciferase assays. Although silencing TUSC2P decreased luciferase activities, silencing Dicer reversed the effects; n =4, ** P <0.01 analysed by t -test, error bar, s.d. ( f ) HaCaT cells were transfected with TUSC2P siRNA combined with or without Dicer1 siRNA. TUSC2P was silenced even in the presence of Dicer1 siRNA; n =4, ** P <0.01 analysed by t -test, error bar, s.d. ( g ) Transfection of 4T1 cells with TUSC2P, TUSC2, TIMP2 and TIMP3 decreased cell migration; n =4, ** P <0.01 analysed by t -test, error bar, s.d. ( h ) Transfection of HaCaT cells with siRNA targeting endogenous TUSC2P increased cell migration. Combined transfection with TUSC2, TIMP2 or TIMP3 partially, but significantly, reversed the effect of TUSC2P on cell migration; n =4, ** P <0.01 analysed by t -test, error bar, s.d. ( i ) Transfection of 4T1 cells with TUSC2P decreased cell migration, which could be partially, but significantly, reversed by transfection with siRNAs targeting TUSC2, TIMP2 or TIMP3; n =4, * P <0.05, ** P <0.01 by t -test, error bar, s.d. Full size image The effects of all related transcripts were tested in cell migration assay. 4T1 cells were transfected with TUSC2P, TUSC2, TIMP2, TIMP3 or a control vector. It was found that transfection with these expression constructs decreased cell migration as compared with the control ( Fig. 9g ). HaCaT cells were also transfected with TUSC2P siRNA and rescued with TUSC2, TIMP2 and TIMP3. Although silencing TUSC2P enhanced cell migration, we found that expression of TUSC2, TIMP2 or TIMP3 significantly reversed the effects of TUSC2P transfection ( Fig. 9h ). In another set of experiments, 4T1 cells stably transfected with TUSC2P or a control vector were transfected with siRNAs targeting TUSC2, TIMP2 or TIMP3. Although the expression of TUSC2P decreased cell migration, silencing of TUSC2, TIMP2 or TIMP3 significantly reversed the effects of TUSC2P ( Fig. 9i ). The effects of TIMP2 and TIMP3 were further tested. 4T1 cells stably transfected with TUSC2-UTR construct were treated with siRNAs targeting TIMP2 or TIMP3. After confirming silencing of TIMP2 and TIMP3 ( Supplementary Fig. S7a ), cell migration was monitored. Silencing TIMP2 and TIMP3 increased cell motility ( Supplementary Fig. S7b ). It was found as well that siRNA-TIMP2 and siRNA-TIMP3 cells invaded through Matrigel-coated transwell membranes faster than the TUSC2-transfected cells ( Supplementary Fig. S7c ). In cell attachment assay, it was found that the siRNA-TIMP2 and siRNA-TIMP3 cells had a decreased rate of attachment and spreading compared with the control cells ( Supplementary Fig. S7d ). Fluorescence-activated cell sorting analysis in the siRNA-TIMP2- and siRNA-TIMP3-treated cells showed decreased cell apoptosis compared with the control ( Supplementary Fig. S7e ). In summary, our results show that the TUSC2P pseudogene can bind to and antagonize endogenous miRNAs, thereby modulating TUSC2, TIMP2 and TIMP3 ( Supplementary Fig. S8a , right side). In the absence of TUSC2P, canonical miRNA signalling mediated through RNA-induced silencing complex can bind and inhibit the translation of TUSC2, TIMP2 and TIMP3 mRNAs ( Supplementary Fig. S8a , left side). The levels of miRNAs were unaffected by TUSC2P transfection ( Supplementary Fig. S8b ), whereas transfection with our six miRNAs of interest increased miRNA levels in the cells ( Supplementary Fig. S8c ). This confirmed effective processing of the miRNA biogenesis pathway. Interestingly, transfection with miRNAs was found to weakly decrease TUSC2P levels ( Supplementary Fig. S8d ). The precise effect of this downregulation awaits further investigation. In a variety of cancer cell lines, it has been reported that TUSC2 mRNA transcripts were detected by northern blot analysis even though there was no TUSC2 protein present [28] , [29] , [30] . This led us to believe that the TUSC2 protein was commonly downregulated by alternative mechanisms. One such option was regulation by miRNAs. Previously, our lab showed that miR-378 was able to bind and inactivate TUSC2 mRNA transcripts [4] . Furthermore, Du et al. [31] showed that miR-93, miR-98 and miR-197 were also capable of binding to the TUSC2 3′-UTR. Here we show that other miRNAs, miR-17, miR-299-3p, miR-520a, miR-608 and miR-661 were also able to bind to the TUSC2 3′-UTR. In this study, we tried to simulate the naturally occurring pseudogene phenomena, initially reported for PTENP1 (ref. 32 ) and later termed as the competing endogenous RNA model. Pseudogenes have been discovered in equal abundance to functional genes and therefore represent a large component of the genome. The human genome has been estimated to have ~20,000 putative pseudogenes [33] . Previously, pseudogenes were classified as ‘junk DNA’ based on the fact that they did not code for proteins. However, it has been recently shown that certain pseudogenes have important roles in maintaining homeostasis, specifically as modulators of miRNAs. This was recently described by Poliseno et al. [32] , where a phosphatase and tensin homologue (PTEN) pseudogene, PTENP1, was discovered to regulate PTEN cellular levels and suppress cell growth. Furthermore, Chin et al. [34] found that single-nucleotide polymorphism variations located in miRNA binding sites of the 3′-UTR could affect miRNA target expression and function. The 3′-UTR of KRAS contained a single-nucleotide polymorphism correlated with an increased risk of non-small cell lung cancer [34] . This single-nucleotide change altered let-7 binding, which resulted in the overexpression of KRAS in lung cancer. A muscle exclusive ncRNA, Linc-MD1, was found to increase the expression of MAML1 and MEF2C, stimulating muscle-specific gene expression by regulating miR-133 and miR-135 activities [35] . Thus, these observations showed that certain pseudogenes perform integral functions in maintaining homeostasis, specifically as modulators of miRNAs. We have reported our findings in the overexpression of the 3′-UTR of versican, CD44 and nephronectin [8] , [9] , [16] . Recently, we also communicated our observations of the competing endogenous RNA functions of versican in liver cancer [36] . Here we continue our hypothesis describing the overexpression of the TUSC2 3′-UTR and TUSC2P in antagonizing multiple miRNAs that endogenously occur in the 4T1 and MB231 cells. The homology between the 3′-UTR of TUSC2 and a potential pseudogene, TUSC2P, was compared. The high degree of similarity (89%) between the two sequences confirmed that the same miRNA binding sites existed in the 3′-UTRs of TUSC2 and TUSC2P. Decreased transcription rates of TUSC2P in cancer cell lines compared with normal cell lines inferred that TUSC2P transcription is lost during malignant transformation. Expression of TUSC2P in breast cancer cell lines isolated from females indicated that the sequence found in chromosome X, which shared 99% homology with the pseudogene TUSC2P expressed by chromosome Y, is actually another pseudogene and can be transcribed. It is anticipated that one copy of these tentative pseudogenes in chromosome X is inactive, whereas male can express two copied of TUSC2P pseudogenes. This would increase the potential loss of TUSC2P in females, especially in a cancerous state. Interestingly, we also detected low levels of TUSC2P expression in prostate cancer cell lines isolated from males. The mechanisms by which expression of TUSC2P is decreased or degradation of TUSC2P is increased await further investigation. The transfection of TUSC2P into 4T1 and MB231 cells elicited similar phenotypic changes as the TUSC2 3′-UTR. Relative to control and TUSC2 coding cells, TUSC2P and TUSC2 3′-UTR transfection was found to relieve transcriptional inhibition on endogenous TUSC2, TIMP2 and TIMP3, thereby increasing their protein levels. Subsequent phenotypic changes were observed in the TUSC2 3′-UTR- and TUSC2P-transfected tumour cells in both 4T1 and MB231 cell lines. TUSC2P and TUSC2 3′-UTR cells had an increased percentage of apoptotic cells, showing increased cell death. This is correlated with the current knowledge of TUSC2 , widely believed to be a tumour suppressor gene that is frequently inactivated during malignant transformation. Overexpression of the TUSC2 3′-UTR also resulted in alterations to the extracellular matrix. There was a decreased migratory and invasive capacity in the TUSC2P and TUSC2 3′-UTR cells compared with the control cells. The variations in these extracellular matrix properties were a result of changes to TIMP2 and TIMP3 expression. We observed an increase in TIMP2 and TIMP3 protein levels in both TUSC2P- and TUSC2 3′-UTR-transfected 4T1 cells and tumours. The TUSC2P and 3′-UTRs of TUSC2, TIMP2 and TIMP3 contain multiple miRNA binding sites in common. By luciferase assay, we confirmed that these miRNA were indeed translational inhibitors of TUSC2, TIMP2 and TIMP3. siRNA targeting TUSC2P were used to confirm the functions of TUSC2P. siRNAs were found to reverse the observed functions of TUSC2P and these results confirmed that the phenotypic changes in the cells were due to the exogenous expression of TUSC2P. The mouse cell line 4T1 does not express transcript with significant homology to TUSC2P. The acquired functions in 4T1 cells transfected with TUSC2P were abolished by retransfection with siRNAs targeting TUSC2P, confirming the observed functions of TUSC2P. The functions of endogenous TUSC2P were also confirmed by siRNAs targeting TUSC2P in HaCaT cells that expressed high level of endogenous TUSC2P. Corroboration of TUSC2P regulating miRNA effect was further confirmed by miRNA transfection. The miRNAs of interest were exogenously overexpressed by transfection into TUSC2P-expressing 4T1 cells. This was done to test miRNA function with the phenotypic changes in the TUSC2P 4T1 cells. miRNA overexpression reversed the observed phenotype of TUSC2P-transfected cells. There was an increase in cell survival, migration and invasion after the exogenous miRNAs were transfected into the TUSC2P 4T1 cells and the HaCaT cells. These experiments indicated that TUSC2P could regulate the functions of miRNAs in a similar manner to the TUSC2 3′-UTR. Investigations into ncRNAs are important because of the complex interactions that these sequences have in comparison with those induced by a single miRNA or gene. The pseudogene, as well as the 3′-UTR, can function as both a modulator of miRNA function and as a mediator of miRNA regulation. As multiple miRNAs can interact with a single ncRNA, these can be important tools, either as buffers or as combinatorial regulators of miRNA. This concept lends itself to the further investigation of ncRNA as functional miRNA inhibitors. The majority of breast-cancer-related deaths are due to metastatic disease. Thus, identifying new targets for metastatic disease progression would greatly improve cancer mortality rates. The 3′-UTRs of TUSC2 and TUSC2P are candidate targets for tumour metastasis due to their ability to reduce cell survival and also inhibit cell migration and invasion. Through its ability to bind multiple miRNAs that are shared in common with TIMP2 and TIMP3, TUSC2P can decrease cell migration and invasion of metastatic breast cancer cells. Thus, the 3′-UTR of TUSC2 and TUSC2P can have a diverse role in fine-tuning gene expression for the inhibition of cancer progression. Further analysis of this non-coding transcript should be investigated for application towards developing cancer therapeutics. Construct generation The pcDNA3.1-TUSC2 3′-UTR construct was created using the 3′-UTR of TUSC2 previously made in the lab, which is also named as Fus-1 (ref. 4 ). The TUSC2 3′-UTR fragment and the TUSC2P fragment were amplified and digested with restriction enzymes Nhe I and Apa I and inserted into Nde I and Apa I opened pcDNA3.1 vector. The protein expression construct of the coding region of TUSC2 was generated previously in the lab [4] . Cell survival assays For survival assays, cells were seeded at the density of 2 × 10 5 cells per well in six-well plates in culture medium (2 ml) containing fetal bovine serum (FBS). After 24 h, cells were washed twice with PBS and then incubated in serum-free medium. After 8 days, the cells were collected and the viable cells were counted after Trypan blue staining. For Annexin V apoptosis assays, the cells were grown in low serum (1%) or serum-free medium for 5 days. The cells were separately washed twice with cold PBS and stained with binding buffer containing fluorescein-labelled Annexin V and with propidium iodide (PI; APC Annexin V Apoptosis Detection Kit I, BD Pharmingen) following manufacturer’s instructions. The cells that were positive for apoptosis (APC annexin V positive, PI negative or APC annexin V positive, PI positive) were analysed by flow cytometry. Cell migration Cells (3 × 10 5 ) were seeded in each well of a six-well plate. The cell cultures were scratched using a 200-μl pipette tip. The cultures were washed with PBS to remove cell debris and the culture media was replaced with serum-free media. Cell migration was monitored and photographed. Distance travelled from the initial scratch site was measured and the migration distance was quantified as described [37] . Cell invasion Cell transwell membrane inserts were placed in 24-well plates and coated with 100 μl of Matrigel that had been diluted (1:10-fold). Cells (1 × 10 3 ) were placed in serum-free media inside the inserts, while media supplemented with 10% FBS was placed at the bottom of the inserts and in the wells of the plates. Cells were incubated at 37 °C and allowed to invade and migrate through the Matrigel and the membrane pores in the inserts. After 20 h, the upper Matrigel layer and cells were removed, while the cells on the surface of the lower side of the membrane were fixed and stained. Cells that migrated onto the lower surface were counted from representative areas for quantification. RNA analysis Expression of the TUSC2 3′-UTR or TUSC2P was confirmed by real-time PCR. In brief, total RNA was extracted from cell cultures using the mirVana miRNA Isolation Kit (Ambion) according to the manufacturer’s instructions. Real-time PCR was performed as previously described [38] . The primers for TUSC2 3′-UTR were previously used in our lab [38] . The primers used as the real-time PCR controls were human-U6RNAf and human-U6RNAr. All primer sequences are provided in the Supplementary Information ( Supplementary Fig. S8e ). siRNA assays Three different siRNA sequences complementary to TUSC2P were used for knocking down TUSC2P: siRNA1: 5′-GUGGUUCAGUCCUGUGAUATT-3′ and 5′-UAUCACAGGACUGAACCACTT-3′; siRNA2: 5′-GCUGUUGUUUGCUACUUAATT-3′ and 5′-UUAAGUAGCAAACAACAGCTT-3′; siRNA3: 5′-GUGGAUGCUUGUGUCUAUATT-3′ and 5′-UAUAGACACAAGCAUCCACTT-3′. The TUSC2P 4T1 cells were seeded at the density of 2 × 10 5 cells per well in six-well plates in 2 ml culture medium containing 10% FBS. Cells were washed twice with serum-free medium 24 h after the inoculation, followed by transfection with the three different siRNAs using Lipofectamine 2000 (Invitrogen). The cells were collected by exposure to trypsin 48 h after the transfection and then subjected to various assays. Tumour formation assay Six-week-old female Balb-c strain nude mice (Jackson Laboratories) were subcutaneously injected with TUSC2-UTR or TUSC2P cells (4T1) and control cells (1 × 10 5 cells). Tumours were retrieved by the end of third week and fixed in 10% formalin, processed, embedded in paraffin and sectioned for immunohistochemistry [39] . The animal use protocol was approved by the Animal Care Committee at Sunnybrook Research Institute. Immunohistochemistry Immunohistochemistry was performed on the paraffin-embedded tissue sections. The tumour sections were processed for antigen retrieval, blocked with 10% goat serum and incubated with primary antibodies against TUSC2, TIMP2 and TIMP3 in tris-buffered saline (TBS) containing 10% goat serum overnight. The sections were then washed and labelled with biotinylated secondary antibody, followed by avidin-conjugated horseradish-conjugated peroxidase provided by the Vectastain ABC kit (Vector, PK-4000). The staining was developed according to the manufacturer’s instructions. The slides were subsequently stained with Mayer’s haematoxylin for counterstaining followed by slide mounting. Western blotting Western blotting was performed on cell and tissue lysates. Briefly, cells were seeded onto a six-well plate at 2 × 10 5 cells per well overnight. They were then transfected with 1 μg of TUSC2-UTR, TUSC2P or the control vector to create stable cell lines. In addition, the TUSC2-UTR and TUSC2P cells were transfected with siRNA against TUSC2-UTR and TUSC2P, respectively, transfected with or different miRNA mimics. The control was a scramble RNA provided in the kit. Proteins were extracted 48 h after transfection by lysing in 60 μl lysis buffer containing protease inhibitors (150 mM NaCl, 25 mM Tris-HCl, pH 8.0, 50 mM EDTA, 20% Triton X-100, 8 M Urea, and 1 × protease inhibitor cocktail). Tissues were weighted and grinded in a quantity of lysis buffer according to weight. All samples were subjected to SDS–PAGE and then transferred to nitrocellulose membranes followed by incubating with antibodies against TUSC2 (Abcam, Ab70182), TIMP2 (Abcam, Ab1828) or TIMP3 (Abcam, Ab58804) at a dilution of 1:500 at 4 °C overnight. Appropriate secondary antibodies were used at 1:2,000 dilutions to incubate with the membranes at room temperature for 2 h. After detection of the protein bands, the blots were stripped and reprobed with mouse monoclonal antibody against β-actin (A5316, Sigma) to confirm equal sample loading. After secondary antibody incubation, the blot was washed and detected using ECL kit (Millipore) in autoradiography. Representative full-gel bots are provided in the Supplementary Information ( Supplementary Fig. S9 ). Luciferase activity assays Luciferase activity assays were performed using a dual-luciferase reporter system developed by Promega (E1960). In brief, 4T1 cells were seeded onto 24-well tissue culture plates at a density of 3 × 10 4 cells per well in the medium containing 10% FBS for 24 h. The cells were co-transfected with the luciferase reporter constructs, corresponding miRNA mimics and Renilla luciferase construct by Lipofectamine 2000. The cells were then lysed using 100 μl of passive lysis buffer per well on a shaker for 30 min, and the lysates were centrifuged for supernatant collection. Twenty microlitres of the supernatants was then mixed with 100 μl of LAR II and then firefly luciferase activities were measured using a luminometer. For the internal control, 100 μl of Stop & Go reagent was added to the samples. Renilla luciferase activities were then measured in the same tube. Luciferase activities between different treatments were compared after normalization with Renilla luciferase activities. The miRNAs were used at a concentration of 100 nM. For the TUSC2 3′-UTR competition experiments, the same luciferase system was used. Cell were transfected with 10 μg of luciferase construct containing TIMP2 or TIMP3 3′-UTR in each well. The cells were also transfected with TUSC2 3′-UTR or the control vector at a concentration of 10 μg plasmid per well. Statistical analysis The results (mean values ±s.d.) of all experiments were subject to statistical analysis by t -test. A P -value <0.05 was considered significant. How to cite this article: Rutnam, Z. J. et al. The pseudogene TUSC2P promotes TUSC2 function by binding multiple microRNAs. Nat. Commun. 5:2914 doi: 10.1038/ncomms3914 (2014).